In operandotracking phase transformation evolution of lithium iron phosphate with hard X-ray microscopy The delithiation reaction in lithium ion batteries is often accompanied by an electrochemically driven phase transformation process. Tracking the phase transformation process at nanoscale resolution during battery operation provides invaluable information for tailoring the kinetic barrier to optimize the physical and electrochemical properties of battery materials. Here, using hard X-ray microscopy—which offers nanoscale resolution and deep penetration of the material, and takes advantage of the elemental and chemical sensitivity—we develop an in operando approach to track the dynamic phase transformation process in olivine-type lithium iron phosphate at two size scales: a multiple-particle scale to reveal a rate-dependent intercalation pathway through the entire electrode and a single-particle scale to disclose the intraparticle two-phase coexistence mechanism. These findings uncover the underlying two-phase mechanism on the intraparticle scale and the inhomogeneous charge distribution on the multiple-particle scale. This in operando approach opens up unique opportunities for advancing high-performance energy materials. Electrochemically driven phase transformation directly influences electrode performance in lithium ion batteries. Advancing our understanding of the mechanism necessitates the development of advanced tools with in operando capability to track the dynamic phase and structural changes of battery materials. This is particularly crucial for olivine-type cathodes, which are representative of a two-phase mechanism but with widely debated specific models. As LiFePO 4 was first reported by Pahdi et al. [1] as a high safety cathode material due to its unique crystal structure, numerous studies have been performed on this promising battery material [2] , [3] , [4] , [5] . Despite the great success in performance and commercialization [6] , [7] , [8] , [9] , the fundamental phase transformation mechanisms accompanying the delithiation process in LiFePO 4 are still actively debated and require in operando studies to come to a consensus. As for large-scale delithiation behaviour (on the multiple-particle scale), most measurements integrate the average information from the entire electrode, overlooking the possible interparticle effect and local region difference [10] , [11] . In addition, most conventional tools only specialize in revealing the structural and compositional information without chemical mapping or imaging capability, lacking effective spatial resolution information [12] , [13] . As a result, the homogeneous and concurrent phase transformation on the multiple-particle scale has become increasingly inadequate. For example, based on theoretical calculation, a new multiple-particle delithiation mechanism was recently suggested where LiFePO 4 particles were delithiated sequentially, not concurrently [14] . In addition to the insufficient understanding of the multi-particle mechanism, more disputes focus on the single-particle delithiation model. Several classic models such as core-shell [1] , [15] , domino cascade [16] , spinodal decomposition [17] and the single-phase kinetic model [18] have been previously proposed to explain the phase transformation process in single-particle scale. Most of these possible models were subsequently confirmed with experimental and theoretical calculated results. For example, the domino-cascade model was confirmed experimentally with LiFePO 4 /FePO 4 precession electron diffraction [19] . The shrinking-core mechanism was also developed by a mathematical model [20] . On one hand, the above conflicting mechanisms and disagreement may be attributed to confusion over the specific experimental condition. On the other hand, these different models for the single-particle delithiation mechanism are mainly based on an entire electrode, assuming that multi-particle behaviour also applies to single-particle systems. In fact, the free energy and phase transition voltage varies with each individual particle, which makes them have different behaviour from the entire electrode [21] . To explore the widely debated mechanism stated above, some advanced techniques (for example, in situ ) have been applied in recent years to understand and examine the dynamic phase transformation in a real battery electrode as it cycles [22] , [23] , [24] , [25] . With a synchrotron X-ray diffraction (XRD) technique, Ogumi and colleagues [22] directly detected a metastable crystal phase of Li x FePO 4 during electrochemical phase transformation under non-equilibrium conditions (at high rate of 10C). However, as discussed above, most conventional in situ synchrotron X-ray technologies are performed with low spatial resolution on an entire electrode. More recent ex-situ work observed the intercalation pathway in many LiFePO 4 particles (partial charged LiFePO 4 , 50% state-of-charge) with scanning transmission X-ray microscopy and found that almost all the LiFePO 4 particles were either completely lithiated or delithiated [23] . Nevertheless, the ex-situ mapping work lacks the dynamic observation and may miss some important information during the fast phase transformation in LiFePO 4 . Recently, in situ conventional X-ray absorption spectroscopy has been used to provide important chemical mapping information to study the redox reaction in LiFePO 4 (refs 26 , 27 ). However, as the resolution determined by the beam size is about 7–10 μm, and the way to make a map is to scan the sample point by point, it will be difficult to catch real-time reactions. Considering the size range of battery materials (hundreds of nanometres to several micrometres), the ability to image the real-time phase transformation at nanoscale resolution is critical for clarifying the phase transformation mechanism in battery materials. Although an in situ transmission electron microscopy technique may allow for a high-resolution observation, the cell design (open structure, specialized electrolytes, short life time, complex operation and so on) does not adequately simulate the real battery operating conditions. In attempting to develop a real-time imaging method with both temporal and spatial resolution precision for battery materials, we face many technical challenges and experimental difficulties. In this work, we overcome those challenges and successfully perform an in operando observation of the delithiation process in multi- and single-LiFePO 4 systems. We use newly developed full-field transmission X-ray microscopy (TXM) at nanoscale resolution combined with X-ray absorption near-edge spectroscopy (XANES) at the National Synchrotron Light Source [28] , [29] . With this unique in operando TXM-XANES approach and the direct map of the inhomogeneous phase distribution for the multi-particle LiFePO 4 system, we disclose the rate dependent inhomogeneity behaviour, which provides more insight into developing high-rate battery technology. As for the single-particle system, our in operando imaging work for the first time presents direct evidence of two-phase coexistence and suggests the two-phase dynamic model in individual LiFePO 4 particles, clarifying the widely debated delithiation mechanisms. Full-field transmission X-ray microscopy Although our recent work [30] and work by Ebner et al. [31] used X-ray attenuation coefficients to quantify the phase transformation within individual particle in three dimensions, the most ideal analytic technique for chemical status identification is XANES. XANES is strongly sensitive to oxidation states and the coordination chemistry of the absorbing element. As a highly element-specific spectroscopy, XANES allows us to detect fine structural and chemical information changes, which is particularly effective to track the nanoscale interfacial phase transformation details. Significantly different than a conventional XANES chemical mapping study [26] , [27] , each pixel of the sample image in our experiment produces the XANES spectrum without scanning the sample. This full-field TXM-XANES imaging produces 2 k by 2 k (for example, a 2K × 2K detector) XANES spectra to provide a full chemical map while at the same time keeping both time resolution(second) and spatial resolution (nanometer). Another unique capability of our in operando TXM-XANES approach is that this method is highly suitable for the versatile coin cells; thus, it enables studies under real battery operation conditions and avoids complex cell design [29] . In addition, the combination of imagery and chemical information using the large field of view (40 × 40 μm) mode enables the mapping of the dynamic phase change evolution in both multi-particle (inter-particle) and single-particle (intra-particle) systems without sacrificing spatial resolution. In our experiments, carbon paper was used as the electrode support to allow better X-ray penetration and enable high-quality imaging ( Supplementary Fig. 1 ). During the phase transformation, chemical information was obtained with TXM-XANES imaging, which was achieved by collecting a series of images at different energies across the absorption edge at each stage under in operando electrochemical conditions. The reference spectra (LiFePO 4 and FePO 4 ) were obtained from the average information in the standard sample at the large field of view (40 × 40 μm). As the spectra of Fe K edge shown in Fig. 1 , with Fe oxidation from LiFePO 4 to FePO 4 in the delithiation process, a clear shift occurs at the absorption edge, which is consistent with previous literature [32] , [33] . After collecting the XANES data at each electrochemical stage, while fitting with the linear combination of the two reference spectra, chemical phase information at each pixel can be obtained. A lens-coupled scintillator with a 2,048 × 2,048 pixel camera detector was used to record images, which can create a chemical phase map when combined with all the chemical information at each pixel [29] . 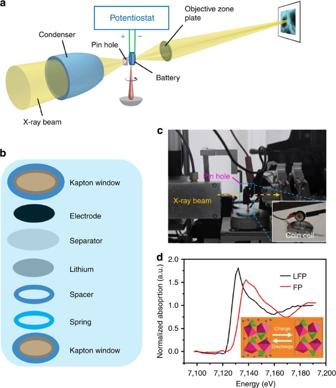Figure 1: Schematic illustration. (a) The principle of full-field transmission X-ray microscopy at X8C beamline, National Synchrotron Light Source. (b) Coin cell parts forin operandoelectrochemical experiment at X8C beamline. (c) The photo image ofin operandoelectrochemical measurement at X8C. (d) The XANES spectra of standard LiFePO4and FePO4(the olivine structures were reproduced with permission from ref.9). Figure 1: Schematic illustration. ( a ) The principle of full-field transmission X-ray microscopy at X8C beamline, National Synchrotron Light Source. ( b ) Coin cell parts for in operando electrochemical experiment at X8C beamline. ( c ) The photo image of in operando electrochemical measurement at X8C. ( d ) The XANES spectra of standard LiFePO 4 and FePO 4 (the olivine structures were reproduced with permission from ref. 9 ). Full size image Chemical mapping of multi-particle LiFePO 4 system We performed our in operando study on LiFePO 4 samples with two size scales. An actual battery electrode is an assembly of many particles with possible particle overlap. In our study, we selected a nano-sized LiFePO 4 sample (200–300 nm) with possible particle overlap to reveal the true electrode feature (multi-particle system), allowing study of the multi-particle delithiation mechanism to elucidate the behaviour of the entire electrode. Meanwhile, to enable a clear observation of the phase transformation in individual particles, we used a micro-sized LiFePO 4 sample (low loading, thin electrode thickness and high conductive carbon ratio) without particle overlap to clarify the delithiation model in a single-particle scale. Previous theoretical studies predicted a single-phase transformation pathway under a non-equilibrium state [18] . Suppression of phase separation was also suggested at high-rate conditions with the simulation method [34] . A recent experimental report with an XRD technique proposed that the phase transformation pathway via a metastable crystal phase only occurs at a high charging rate condition [22] , in contrast to the other study with XANES detecting only pure phase (LiFePO 4 or FePO 4 ) with a half-charged electrode [23] . Thus, the phase transformation process in LiFePO 4 may be rate-related. Accordingly, in our electrochemical measurements, two rates of 0.1C (it takes 10 h to fully charge the electrode) and 5C(it takes 0.2 h to fully charge the electrode) were used to examine the phase transformation process. First, we performed our study on a representative region (a large field of view, 40 × 40 μm) of the nano-LiFePO 4 electrode (multi-particle system) to understand the dynamic process within the entire electrode. The delithiation reaction at a high rate of 5C was first tracked by TXM-XANES imaging approach. 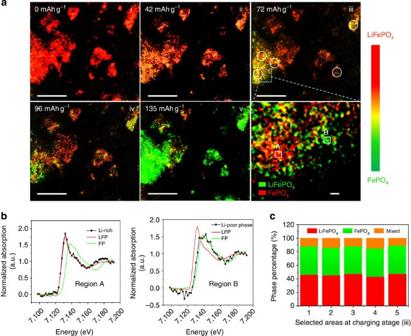Figure 2:In operando2D chemical mapping of multi-particle LFP system at a fast charging rate of 5C. (a) Two-dimensional chemical mapping; (b) XANES at selected regions (square A and B) at charging stage iii; (c) histograms of statistical analysis of phase compositions at five selected regions (round zones) at charging stage iii. Scale bar: 10 μm for the five 2D maps, 200 nm for the enlarged map. Figure 2 shows the composition and two-dimensional (2D) chemical mapping at the phase transformation process in the multi-particle system during the fast delithiation process (see charging profile in Supplementary Fig. 2 ). The 2D phase composition maps in Fig. 2a provide the spatial distribution information of large-area (40 × 40 μm 2 ) particles during the charging process. The phase map obtained at the fresh sample indicated the pure phase of LiFePO 4 (red) zone in these particles. With charging, the in operando 2D chemical phase maps show a continued phase transformation from LiFePO 4 (red) to FePO 4 (green) during the fast charging process. At the end of the charging process, most of the LiFePO 4 particles were transformed to FePO 4 (green). Figure 2: In operando 2D chemical mapping of multi-particle LFP system at a fast charging rate of 5C. ( a ) Two-dimensional chemical mapping; ( b ) XANES at selected regions (square A and B) at charging stage iii; ( c ) histograms of statistical analysis of phase compositions at five selected regions (round zones) at charging stage iii. Scale bar: 10 μm for the five 2D maps, 200 nm for the enlarged map. Full size image The overall phase transformation information can be obtained by the average XANES spectra shown in Supplementary Fig. 3 , which is consistent with numerous previous studies from XRD and XANES, indicating the phase transformation from LiFe 2+ PO 4 to Fe 3+ PO 4 . Surprisingly, as shown in these 2D maps in Fig. 2a , phase transformation spatial distribution at each stage is not homogeneous. During the charging process, two phases (LiFePO 4 and FePO 4 phase zones) were found to coexist within the electrode. During the second charging stage, minor particles were completely changed to FePO 4 phases, and coexist with major intact LiFePO 4 particles. As charging continues, more and more pure FePO 4 phases were formed, but still some LiFePO 4 phases were kept intact. This phenomenon is more remarkable at the third charging stage. After enlarging the region (square zone at Fig. 2a, iii ) from the third stage of the sample, the 2D map shows few mixed phase zones (yellow). Instead, the phase is either fully lithiated LiFePO 4 (red) or fully delithiated FePO 4 (green). The XANES spectra obtained at the small region A and B correspond to a nearly pure LiFePO 4 and FePO 4 phase, respectively, indicating the inhomogeneity of phase distribution. More statistics taken over a large region during the fast charging process are shown in Supplementary Fig. 4 . The histogram of phase composition further confirms that with the fast charging process, the majority of these LiFePO 4 particles completely transform to delithiated FePO 4 without the intermediate mixed phase process. These quantitative results show that two phase zones coexist within a multi-LiFePO 4 system during the delithiation process. In other words, this dynamic observation of the delithiation process indicates that at a fast rate, the intercalation pathway within many LiFePO 4 particles is not concurrent. The inhomogeneity in the delithiation process happens in multi-particle LiFePO 4 systems at a high charging rate. Contrary to the intercalation pathway within the multi-particle LiFePO 4 system at high rates, low-rate charging shows ‘concurrent’ intercalation pathway. 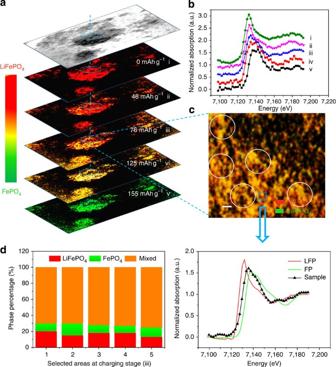Figure 3:In operando2D chemical mapping of multi-particle LFP system at a slow charging rate of 0.1C. (a) Two-dimensional chemical mapping; (b), average XANES spectra; (c) enlarged chemical map of the selected area at the charging stage iii; (d) histograms of phase composition at five selected regions (round zones inc) and the XANES of the selected region (blue square zone inc). Scale bar: 200 nm for the enlarged map. Figure 3 shows the phase transformation and 2D chemical phase mapping information for a multi-particle LiFePO 4 system at a low charging rate of 0.1C. The low charging rate resulted in a higher charging capacity of 155 mAh g −1 . Similar to the above result at the fast charging rate, the 2D maps ( Fig. 3a ) and the average XANES spectra ( Fig. 3b ) at the slow charging rate reveal a continuous phase transformation process. However, contrary to the fast charging multiple-particle LiFePO 4 system, the 2D chemical phase maps at the slow charging rate show homogeneous phase distribution at each charging stage, which can be more clearly observed in the enlarged maps during the three charging stages ( Fig. 3c and iii, vi and v in Supplementary Fig. 5 ). The histogram of phase composition ( Fig. 3d ) based on the statistical information at the selected regions (round region at Fig. 3c ) shows the phase distribution in the slow charging process is homogeneous (or mixed phase), neither pure LiFePO 4 nor FePO 4 , supporting the homogeneous phase distribution. In other words, at a slow charging rate, the delithiation process in the electro-scale (multi-particle system) is homogeneous, which is further supported by the XANES spectrum shown in Fig. 3e at the selected small region (square area in Fig. 3c ), where it shows a homogeneous phase composition between LiFePO 4 and FePO 4 . Representative XANES spectra for the selected regions and the phase composition based on the fitting result of the two partially charged samples are presented in Fig. 4 . As for the partially fast charged sample ( Fig. 4a ), the phase is either Li-rich Li 1-α FePO 4 (LFP, region 2) or Li-poor Li β FePO 4 (FP, region 1 and 3). By comparison, the three regions at the partially slow-charged sample show a similar phase composition. More quantitative analysis and the corresponding histogram of the phase composition at each charging stage are shown in Supplementary Fig. 6 and Supplementary Table 1 . The above quantitative results suggest that in a multiple LiFePO 4 particle system, phase transforms concurrently at a slow charging rate but proceeds inhomogeneously at a fast rate. The schematic proposing the phase transformation mechanism in a multi-particle LiFePO 4 system is shown in Fig. 5 . Each circle represents an aggregation of particles, not an individual one. Figure 3: In operando 2D chemical mapping of multi-particle LFP system at a slow charging rate of 0.1C. ( a ) Two-dimensional chemical mapping; ( b ), average XANES spectra; ( c ) enlarged chemical map of the selected area at the charging stage iii; ( d ) histograms of phase composition at five selected regions (round zones in c ) and the XANES of the selected region (blue square zone in c ). Scale bar: 200 nm for the enlarged map. 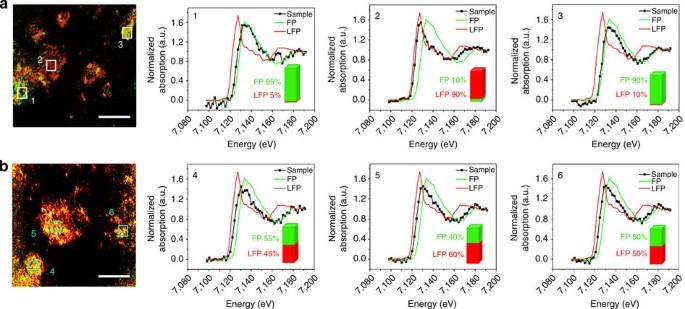Figure 4: Phase composition analysis at partially charged multi-particle LiFePO4system electrodes. (a) The fast charging rate of 5C; (b) the slow charging rate of 0.1C. Scale bar, 10 μm. Full size image Figure 4: Phase composition analysis at partially charged multi-particle LiFePO 4 system electrodes. ( a ) The fast charging rate of 5C; ( b ) the slow charging rate of 0.1C. Scale bar, 10 μm. 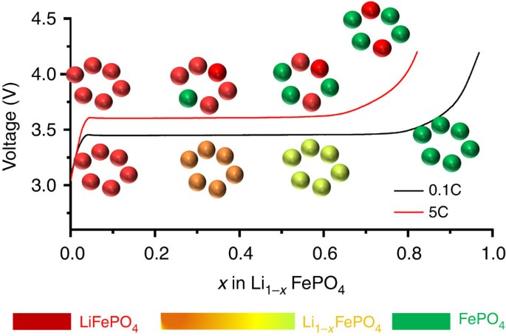Figure 5: Schematic illustration for multi-particle LiFePO4system. Phase transformation mechanism and intercalation pathway at fast and slow charging rates for multi-particle LiFePO4system. Each circle represents a multi-particle nano-LFP aggregation, not single particle. Full size image Figure 5: Schematic illustration for multi-particle LiFePO 4 system. Phase transformation mechanism and intercalation pathway at fast and slow charging rates for multi-particle LiFePO 4 system. Each circle represents a multi-particle nano-LFP aggregation, not single particle. Full size image Chemical mapping of single-particle LFP system In addition to the multi-particle mechanism, understanding single-particle behaviour is critical to clarifying the delithiation mechanism in an intraparticle system to serve for improving their performance. To track the delithiation process in single particle, we selected larger-sized LiFePO 4 sample (micron-sized) to avoid interference caused by particle overlap. The charging profiles at a fast rate (1C) and slow rate (0.02C) for single-particle system were shown in Supplementary Fig. 7 . 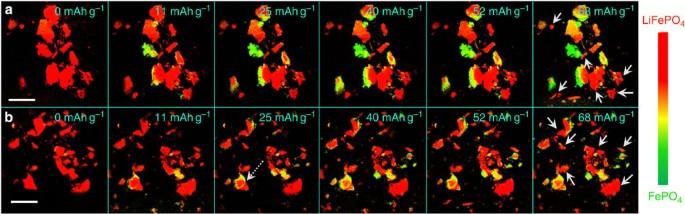Figure 6: Temporal phase transformation evolution in intraparticle at a fast charging rate of 1C. Two randomly selected regions with a large field of view (40 × 40 μm) represent the entire electrode delithiation reaction behaviour. The solid arrows indicate intact particles during the charging process, and the dashed arrows shows the crack formation in some particles due to mismatch and energy release in the two-phase interface. Scale bar, 10 μm. Figure 6a,b shows the 2D chemical phase mapping of LiFePO 4 particles at two randomly selected regions (a large field of view, 40 × 40 μm) during a fast charging process. First, we further observed the inhomogeneity in electrochemical delithiation process at a high rate. Some particles undergo a continuous phase transformation, whereas others keep intact to the end (see arrows in Fig. 6 ). This inhomogeneity delithiation behaviour occurs at these random regions (more results not shown here), indicating that this phenomenon is ubiquitous, which also provide additional experimental evidence of the rate-dependent delithiation inhomogeneity in the above multi-particle system. Second, it is the first time to directly observe the dynamic delithiation evolution in individual LiFePO 4 particles in a conventional coin cell. Interestingly, all these individual particles involve intraparticle two-phase coexistence at this fast charging rate. Similar delithiation behaviour was also found in the slow charging sample ( Fig. 7 ). Different from traditional isotropic ‘core-shell’ model in which the reaction front moves radially inward along multi-directions, [15] the delithiation process and the LiFePO 4 /FePO 4 interface in this work was observed to move only along certain preferential sites. Although it is hard to identify the exact crystallographic direction in specific individual particles due to the irregular particle morphology and size, the statistics information based on the overwhelming majority of the individual particle’s behaviour confirm one-dimensional lithium ion transportation. Furthermore, individual particle behaviour appears to be independent of morphology and size in this study (micron-scale particles). Figure 6: Temporal phase transformation evolution in intraparticle at a fast charging rate of 1C. Two randomly selected regions with a large field of view (40 × 40 μm) represent the entire electrode delithiation reaction behaviour. The solid arrows indicate intact particles during the charging process, and the dashed arrows shows the crack formation in some particles due to mismatch and energy release in the two-phase interface. Scale bar, 10 μm. 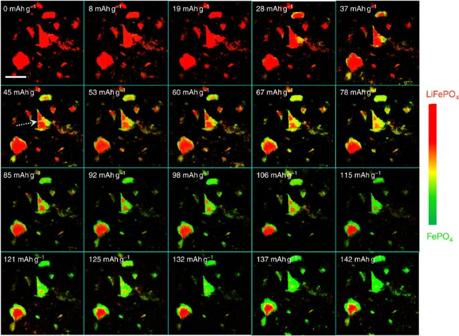Figure 7: Temporal phase transformation evolution in intraparticle at a slow charging rate of 0.02C. The entire electrode shows homogeneous delithiation reaction process and almost all particles undergo the phase transformation process. The dashed arrows reveal cracks formation in some individual particles. Scale bar, 10 μm. Full size image Figure 7: Temporal phase transformation evolution in intraparticle at a slow charging rate of 0.02C. The entire electrode shows homogeneous delithiation reaction process and almost all particles undergo the phase transformation process. The dashed arrows reveal cracks formation in some individual particles. Scale bar, 10 μm. Full size image With clearer observation, the delithiation mechanism in these individual particles can fall into two broader categories, one-site pathway and multi-site parallel-direction transportation. The representative particle of each model and the corresponding schematic illustration are shown in Fig. 8 . As for model a, the delithiation pathway moves almost solely along one site. By comparison, phase transformation may occur at multi-site in model b, but it seems that the delithiation reaction still primarily dominates at certain sites (for example, the top edge in this particle). Furthermore, it is plausible that lithium ion diffusions along these sites are in parallel in model b based on the statistic observation. The variation of Fe 2+ to Fe 3+ oxidation state along the line direction in the XANES line profile at each sample is consistent with the corresponding chemical image map. The phase composition of FePO 4 phase based on the linear combination fitting shows the same trend. 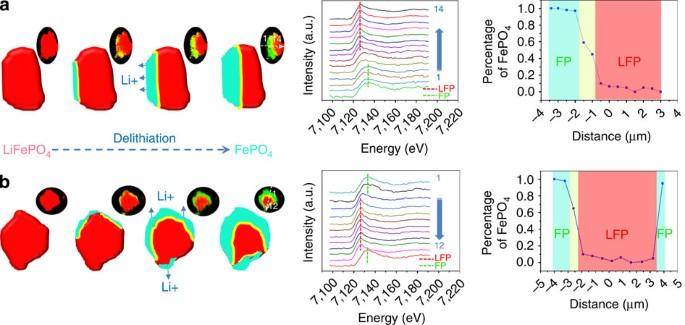Figure 8: Schematic illustration for single-particle LiFePO4system. The modelsaandband the corresponding actual particles represent the two typical delithiation processes revealed byin operandoTXM. Figure 8: Schematic illustration for single-particle LiFePO 4 system. The models a and b and the corresponding actual particles represent the two typical delithiation processes revealed by in operando TXM. Full size image The above in operando studies suggest that the inhomogeneity of phase transformation within multi-particle systems is rate dependent. The inhomogeneity phenomenon was previously reported on the phase distribution along the cross-section direction to the current collector using ex-situ synchrotron X-ray micro-diffraction [35] . Differently, here we found inhomogeneity in the entire electrode with hard X-rays penetrating through the electrode. Using direct imaging technology, our result also confirms the recent charge dynamic study in a LiFePO 4 electrode with soft X-ray spectroscopy that observed inhomogeneity in polymer electrolyte electrodes with low ion conductivity [36] . In our work, the use of low active material loading and liquid electrolyte is supposed to enhance the ionic and electron conductivity. However, the inhomogeneity of phase distribution still happens. Therefore, the observed inhomogeneity at high rates implies an unsolved mystery in the LiFePO 4 electrode. Ideal electrode architecture involves all particles ionically and electronically ‘connecting’ with each other, so that both lithium ions and electrons are equally available to each particle. Therefore, in addition to investigating the conventional solution of size reduction to address the rate performance in individual particle, our in operando study highlights the importance of electrode-scale homogeneity to achieve high rate performance. This refined understanding of the multi-particle LiFePO 4 delithiation mechanism motivates more efforts in optimizing the entire electrode architecture rather than focusing only on battery materials’ individual features to develop a future fast charge/discharge battery. As for the single-particle system, the phase transformation process in these individual particles is similar to the classic anisotropic ‘domino-cascade’ model [16] . Nevertheless, in comparison with the classic model, which is based on nanoscale particles where all individual particles are single phase (predominantly fully delithiated or fully lithiated phase), in our study an intraparticle two-phase coexistence was observed at large particle scale under in operando electrochemical conditions. This first time direct observation and tracking of the two-phase evolution at nanoscale resolution under real battery operation conditions has been executed to clarify and enrich the previous theoretical model. Olivine-type lithium metal phosphates possess a unique polyoxyanionic crystal structure. When electrochemical delithiation starts, the edge-sharing olivine structure restricts the flexibility for solid solution phase formation [37] . Instead, two end-member phases, LiFePO 4 and FePO 4 , dominate the crystalline at the beginning. For small particles, the large structural mismatch and local constraints between the two phases drive the fast boundary displacement, and the elastic energy facilitates the delithiation reaction, leading to a rapid phase transformation process. Thus, a fully delithiated or lithiated single phase was formed at nanoscale particles, which represents the classic ‘domino-cascade’ mode. In contrast, large-sized particles are not so robust that the large mismatch in micron scale particles generally result in energy relaxation [38] , contributing to the emergence of cracks or structural dislocations, as some cracks were often found in many different reports [39] , [40] . In our study, cracks are also found in some individual particles (see dashed arrows in Figs 6 and 7 ). The crack regions show facile phase transformation, as shown in the Figs 6 and 7 , which is in agreement with the previous transmission electron microscopy result that phase boundary migration is severely affected by structural defects. [38] The consequence of the energy relaxation is the decrease of the local constraints, which weaken the driving force for boundary displacement. Furthermore, the wide interfacial region in larger particle may further limit the displacement process (yellow interface region shown in most individual particles in Figs 6 and 7 ) [41] . Therefore, due to these multiple factors, the quick interfacial reaction and boundary displacement in larger particles are not allowed, resulting in the two phases coexisting within large intraparticles. In summary, the phase transformation mechanism and intercalation pathway within multi-particle and individual LiFePO 4 particles during battery operation are investigated with full-field X-ray microscopy technique. As for the multi-particle scale, a rate-dependent phase inhomogeneity mechanism is suggested. At a slow rate, a homogeneous phase distribution indicates that LiFePO 4 particles transform concurrently at the entire electrode. At a high rate, two-phase zones (either fully lithiated LFP or fully delithiated FP) coexist during the phase transformation. The rate-dependent phase inhomogeneity mechanism highlights the importance of maintaining the uniform electrode structure (thickness, porosity, conductive carbon distribution and so on) to improve battery rate performance, rather than focusing solely on the conventional size-reduction strategy. As for single-particle delithiation mechanism, for the first time, we provide a direct experimental evidence of the two-phase coexistence within individual particles at micron scale. These discoveries not only clarify the previous delithiation reaction model, but also provide the fundamental basis for the further development of high-rate two-phase battery materials. In addition, this work demonstrates the unique capability of applying TXM-XANES techniques in understanding battery materials with complex mechanism in a real battery operation condition. This in operando approach has a wide variety of applications in other fields, such as fuel cells, catalysis, environmental science and biological science. Materials and electrochemical measurements LiFePO 4 powder (MTI Corp) was mixed with acetylene black and polyvinylidene fluoride with a weight ratio of 50:35:15 (C:polyvinylidene fluoride:LFP) in N -methyl-2-pyrrolidone solvent to produce the slurry. The resultant slurry, pasted on commercial carbon paper, was dried at 100 °C under vacuum for 24 h to form the working electrode. The coin cells (2032) with Kapton windows were then assembled in a high purity argon-filled glove box using lithium metal as the anode and 1 M LiPF 6 (dissolved in a solvent consisting of 50% ethylene carbonate and 50% dimethyl carbonate by volume) as the electrolyte. The galvanostatic charge–discharge measurement was performed on an electrochemical workstation (Potentiostat/Galvanostat/EIS (VMP3)) at room temperature. In operando TXM study The TXM imaging with hard X-ray was conducted at beamline X8C, NSLS, BNL. A field of view of 40 × 40 μm 2 with a 2 k × 2 k CCD camera was used. The in operando TXM imaging was conducted on the assembled LiFePO 4 coin cell during the delithiation process. To study the chemical state evolution, a full XANES image series was collected at each charging stage during the delithiation process. Each XANES image series was measured by scanning Fe absorption K-edge from 7,089 to 7,189 eV, with 2 eV step size, and one TXM image at one energy step, which generated 1 k × 1 k XANES spectra with 2 × 2 binned pixels. Each image was collected with 10 s exposure time. Camera pixels (2 × 2) were binned into one output image pixel. XANES data analysis All the XANES data analysis was carried out using customized programme (MatLab, MathWorks, R2011b) developed in house (beamline X8C group, NSLS, BNL). Background normalization was carried first out for TXM images, with a unique background image collected at every energy. With all 1,024 × 1,024 pixels, we can extract the full spectrum (X-ray intensity versus energy) for each pixel. Based on Beer’s Law, the attenuation of X-ray from a given phase with attenuation coefficient μ and thickness t can be written as: where I 0 is the incident X-ray intensity and I is the X-ray intensity after the attenuating phase. Notice that μ is a function of energy and can be attributed to two phases: LiFePO 4 and FePO 4 . The scaled −ln(I/I 0 ) at each of the 1,024 × 1,024 pixels was then fitted with the linear combination of three μ -values. The ratio of the weighting factor is an analogy of the thickness fraction and therefore represents their volume fraction. The pixels which do not show significant contrast change before and after the Fe edge (indicating that there is no Fe in those pixels) can be easily excluded through a filtering process. The fitting was carried out by calculating the R value for each spectrum (for each pixel), which is defined as: where E i is 7,089 eV, E f is 7,189 eV, data E is the −ln(l/l 0 ) value for the given pixel at energy E , the ref E is the possible fitting reference −ln(l/l 0 ) value, a linear combination of LiFePO 4 and FePO 4 . We considered all possible combination with LiFePO 4 and FePO 4 by 5 vol. % resolution, which resulted in a total 231 possible combinations. For a given pixel with its associated spectrum, the smallest R was determined to find a best-matched phase combination of LiFePO 4 and FePO 4 that can be assigned to the specific pixel. The standard XANES spectra for the reference materials LiFePO 4 (MTI Corp, USA) and FePO 4 (Sigma, USA) were measured at the TXM beamline X8C (NSLS, BNL). The TXM XANES imaging on the reference materials was carried out by using the same condition as used in the XANES imaging for the LiFePO 4 battery cell sample. The detector used at our beamline is a CCD detector with a Retiga 40DC camera. The noise of the detector is taken care of for each image by a standard ‘dark-field’ subtraction. Multiple dark current images are collected without X-ray to record the noise of the detector (CCD). This is a standard procedure and is done routinely as part of the built-in data collection procedure. In terms of error estimation, first, the data points that do not exhibit sufficient absorption edge jump are rejected. Second, the fitting process involves a calculation of the residual R value (see Methods—XANES Data Analysis). The fitted results that exhibit larger than 0.5% of residual errors are rejected as well. Our result and conclusion are well reproducible based on multi-sample experiments. Specially, as for both single-particle and the multi-particle LiFePO 4 mechanism analysis, we performed the in operando TXM studies on three coin cells for each electrochemical experiment condition (fast charging and slow charging rate). At each coin cell, we randomly selected four to five regions (a large field of view, 40 × 40 μm) for XANES analysis. Owing to the standard electrode preparation and coin cell assembly procedure, all the selected regions at specific electrochemical condition (fast or slow charge) reveal the almost same delithiation feature. In a word, the results and conclusion in this paper are based on the statistical analysis of 12 coin cells (~50 regions with each region of 40 × 40 μm). How to cite this article: Wang, J. et al. In operando tracking phase transformation evolution of lithium ion phosphate with hard X-ray microscopy. Nat. Commun. 5:4570 doi: 10.1038/ncomms5570 (2014).